High-performance hybrid oxide catalyst of manganese and cobalt for low-pressure methanol synthesis Carbon dioxide capture and use as a carbon feedstock presents both environmental and industrial benefits. Here we report the discovery of a hybrid oxide catalyst comprising manganese oxide nanoparticles supported on mesoporous spinel cobalt oxide, which catalyses the conversion of carbon dioxide to methanol at high yields. In addition, carbon–carbon bond formation is observed through the production of ethylene. We document the existence of an active interface between cobalt oxide surface layers and manganese oxide nanoparticles by using X-ray absorption spectroscopy and electron energy-loss spectroscopy in the scanning transmission electron microscopy mode. Through control experiments, we find that the catalyst’s chemical nature and architecture are the key factors in enabling the enhanced methanol synthesis and ethylene production. To demonstrate the industrial applicability, the catalyst is also run under high conversion regimes, showing its potential as a substitute for current methanol synthesis technologies. Carbon dioxide is a harmful greenhouse gas produced in large quantities as a by-product in many industrial processes and in the generation of electricity [1] . In order to decrease emissions and prevent the increase of atmospheric carbon dioxide, carbon-capture technologies have emerged to harvest, store and transport the gas. The efficient utilization of these CO 2 sources to produce fuel or higher-value chemicals is the subject of much research interest, as CO 2 makes an alternative, economical carbon feedstock [2] . An attractive possibility is methanol production: It is an easily transportable fuel; fuel cell technology already exists (direct methanol fuel cells); and it can be used as a precursor for many valuable chemical intermediates. A number of catalytic and electrocatalytic reaction schemes over various catalysts have been documented for the hydrogenation of CO 2 (refs 3 , 4 , 5 , 6 , 7 ). Electrocatalytic and photo-electrocatalytic routes show promise; however, selective reduction of CO 2 to methanol with a low overpotential is difficult [8] , [9] , [10] . Homogeneous systems have been demonstrated, such as iridium catalysts for use in basic aqueous media at elevated pressure [11] , or ruthenium-based single-site organometallic catalysts for hydrogenation of supercritical CO 2 to make formic acid [12] , [13] . Even nonmetal Lewis pairs have been successfully implemented as phase-transfer catalysts to solubilize and reduce CO 2 (refs 14 , 15 ). Heterogeneously, Cu/ZnO supported in Al 2 O 3 catalyses methanol synthesis with selectivity greater than 50% via hydrogenation of CO 2 at high pressures (>20 bar) [16] . More recently, a Ni–Ga heterogeneous catalyst was reported as an alternative to the traditional Cu/ZnO/Al 2 O 3 methanol synthesis [7] . However, there is yet no chemically, catalytically and economically viable substitute for Cu such as to hydrogenate CO 2 to methanol in high yields. In this paper, we report a highly active and highly selective hybrid oxide catalyst composed of manganese oxide nanoparticles (NPs) supported on a mesoporous cobalt oxide support for the production of methanol under mild pressure and temperature conditions. The nature of the interfacial domains of the catalyst is shown to be extremely important, as the activities of the individual catalyst components are lower and less selective to methanol, emphasizing the importance of the hybrid architecture. Catalyst performance Control of activity and selectivity through the formation of specific interfacial domains reveals to be highly efficient in the case of CO 2 hydrogenation to methanol. We obtained 30% methanol selectivity and 0.18 s −1 yield for a hybrid catalyst consisting of MnO x NPs supported on mesoporous Co 3 O 4 (m-Co 3 O 4 ). The turnover frequency (TOF) of this catalyst compared with the support alone (m-Co 3 O 4 ) or the MnO x NPs supported on mesoporous SiO 2 (m-SiO 2 ) is 3 and 25 times higher, respectively. In terms of selectivity, the differences between our hybrid catalyst and its parent components are very pronounced as depicted by Fig. 1b . The cobalt support alone produces 35% of CO, 35% of CH 4 and ∼ 20% of methanol; the MnO x NPs produce primarily CO with a selectivity peaking at 85%. Another unique attribute of this catalyst is its ability for C–C bond formation. In addition to the high methanol yield, the catalyst produces ethylene ( ∼ 10%). 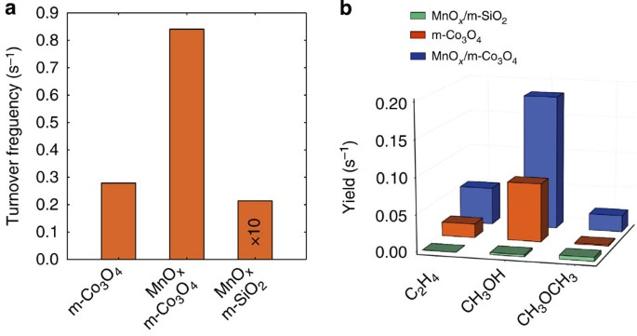Figure 1: Catalytic performance. Results for catalytic measurements carried out on different catalysts. (a) Activity expressed in terms of turnover frequency of the cobalt oxide support, the manganese nanoparticles supported on cobalt oxide and the manganese nanoparticles supported on inert SiO2. (b) Yield of these catalysts towards ethylene, methanol and dimethyl ether. Figure 1: Catalytic performance. Results for catalytic measurements carried out on different catalysts. ( a ) Activity expressed in terms of turnover frequency of the cobalt oxide support, the manganese nanoparticles supported on cobalt oxide and the manganese nanoparticles supported on inert SiO 2 . ( b ) Yield of these catalysts towards ethylene, methanol and dimethyl ether. Full size image Catalyst characterization The reason for its higher activity and better selectivity is linked to the structure of the catalyst that we identify as uniformly distributed grains of metallic cobalt cores with thin cobalt oxide shells in contact with the manganese oxide. This picture was derived from X-ray absorption spectroscopy (XAS) in the total electron yield (TEY) mode and electron energy-loss spectroscopy (EELS) in the scanning transmission electron microscopy (TEM) mode, and will be discussed below. The EELS technique, which gives bulk information, indicates the predominance of metallic cobalt. From a fresh to spent catalyst, the oxygen average for cobalt, plotted as a function of the cobalt L 3 to L 2 edge ratio, goes from 1.4 to 0.3 (see Fig. 2d ). The former value suggests the existence of a spinel cobalt oxide phase (that is, for m-Co 3 O 4 the cobalt to oxygen theoretical ratio is 1.34), whereas the latter confirms a more metallic nature ( ∼ 70%) of the grain. Manganese is only present in 1 weight % and does not alter the conclusions arrived at above. 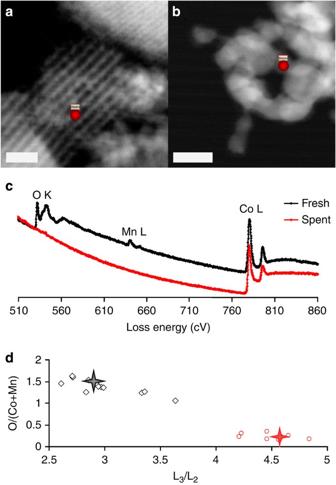Figure 2: EELS characterization. Representative STEM images of (a) the pristine and (b) the spent MnOx/m-Co3O4catalysts. (c) The corresponding EELS point spectra measured from the spots marked with the red dots inaandb. (d) Plots of O/(Co+Mn) versus L3/L2ratios for the pristine (black diamonds) and spent (red circles) catalyst obtained from the EELS analysis. Stars indshow the values averaged over 10 EELS spectra for each catalyst. Scale bars, 50 nm. Figure 2: EELS characterization. Representative STEM images of ( a ) the pristine and ( b ) the spent MnO x /m-Co 3 O 4 catalysts. ( c ) The corresponding EELS point spectra measured from the spots marked with the red dots in a and b . ( d ) Plots of O/(Co+Mn) versus L 3 /L 2 ratios for the pristine (black diamonds) and spent (red circles) catalyst obtained from the EELS analysis. Stars in d show the values averaged over 10 EELS spectra for each catalyst. Scale bars, 50 nm. Full size image Contrastingly, the surface-sensitive XAS in TEY measurement shows the following ( Fig. 3 ): the spinel Co 3 O 4 phase of the support disappeared completely in favour of cobalt (II) oxide (from 0 to 80%; see Supplementary Figs 1 and 2 ); the fraction of metallic cobalt increases as well in the spent catalyst (from 0 to 20%; see Supplementary Fig. 2 ). The complimentary information gained from these techniques indicates that most of the grains are metallic, while the surface appears to be mainly cobalt oxide, leading to the conclusion previously stated of the core/shell grain structure. 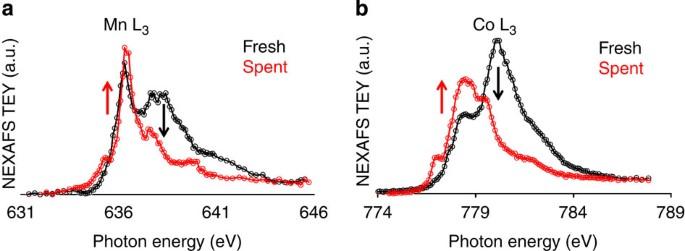Figure 3: XAS characterization. X-ray absorption spectra of (a) manganese L3edge and (b) cobalt L3edge comparing the fresh and spent MnOx/m-C3O4catalysts. The changes in the profile of these spectra evidence the change in the oxidation state for both the Co and Mn. Arrows indicate relative changes in oxidation states. Figure 3: XAS characterization. X-ray absorption spectra of ( a ) manganese L 3 edge and ( b ) cobalt L 3 edge comparing the fresh and spent MnO x /m-C 3 O 4 catalysts. The changes in the profile of these spectra evidence the change in the oxidation state for both the Co and Mn. Arrows indicate relative changes in oxidation states. Full size image Meanwhile, the manganese oxide is also the subject of a reduction from Mn(IV) and Mn(III) to Mn (II). The result shows that the spent NPs are mainly made of MnO with a small amount of spinel oxide (Mn 3 O 4 ). The active catalyst is produced by temperature reduction at 350 °C, and we have investigated the effect of different hydrogen reduction temperatures on the activity of the catalyst. At higher reduction temperature, that is, 450 °C, the catalytic TOF drops ( Supplementary Fig. 3 ), which we cannot link to the change in overall surface area. Instead, we have correlated this drop to the increasing concentration of metallic cobalt at the surface as indicated by XAS ( Supplementary Figs 1 and 2 ). These results evidence the importance of the CoO phase in contact with the MnO x phase. We believe that the existence of a MnO x /CoO interface is paramount to the enhanced activity of the catalyst. A possible explanation is that the presence of manganese NPs helps reduce the CO 2 to CO species, which can further react with surface-layer CoO of the support, responsible for the formation of methanol and chain growth (ethylene). Our hypothesis is based on the fact that the selectivity of the NPs towards CO is extremely high. One would expect the hybrid catalyst’s selectivity towards CO to be additive, whereas the hybrid is even lower than m-Co 3 O 4 alone. To verify our hypothesis, we produced an inverted hybrid catalyst, that is, CoO x NPs supported on mesoporous MnO 2 (m-MnO 2 ). In this case, the activity of the inverted catalyst is dominated by the support, as its selectivity is similar to that of the m-MnO 2 support (that is, both primarily produce CO as indicated in Supplementary Fig. 4 ). These results prove that the architecture and chemical nature of the interface is vital to the activity of a catalyst. Finally, we investigated the industrial applicability of our hybrid catalyst as shown in Fig. 4 . We have compared the catalyst at different conversions under the same conditions (4 bar and 250 °C), demonstrating an even higher selectivity towards methanol than the one observed for low conversion (from 30 to 45%). Previous reports on Cu/ZnO methanol catalysts at high pressures (10–50 atm) show methanol yields on the order of 0.01–0.020 s −1 (refs 16 , 17 ) with variations depending on preparation and pretreatment [18] . Our catalyst has a methanol yield of 0.18 s −1 , approaching a 10-fold increase in activity. In addition, a recent paper reported in ref. 7 provides a yield at comparable pressure conditions to our catalyst of 6 × 10 −5 s −1 . Thus, not only is the MnO x /m-Co 3 O 4 catalyst more active, but compared with current Cu/ZnO methanol catalysts, our hybrid catalyst works under milder conditions, which make it an attractive alternative. The substantial savings in the cost and energy consumption make it an environmentally friendly catalyst in phase with the development of a more sustainable and greener industry. 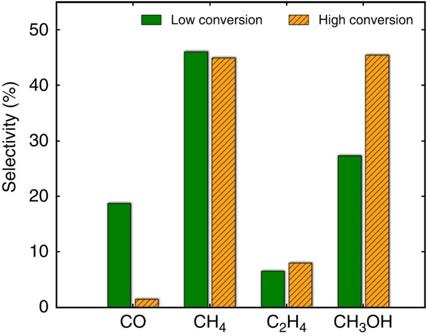Figure 4: Industrial performance. Selectivity of CO, methane, ethylene and methanol at low (solid) and high (hashed) conversion regimes at 250 °C for the MnOx/m-Co3O4catalyst. Figure 4: Industrial performance. Selectivity of CO, methane, ethylene and methanol at low (solid) and high (hashed) conversion regimes at 250 °C for the MnO x /m-Co 3 O 4 catalyst. Full size image In this study, we reported the discovery of a highly active and selective methanol synthesis catalyst comprising MnO x NPs supported in mesoporous cobalt oxide. In addition to methanol, ethylene was produced in modest quantities, indicating carbon–carbon bond formation pathways. On the basis of surface-sensitive XAS and EELS in the scanning TEM mode, we determined the active phase of the catalyst as MnO NPs dispersed over grains of cobalt comprising CoO surfaces with metallic Co cores. The existence of a MnO/CoO interface facilitated an activity enhancement towards methanol synthesis, compared with the separate NPs and supports. The importance of the nature and architecture of the interfacial domains was highlighted by the use of an inverted catalyst. Moreover, catalytic runs under high conversion regimes demonstrated potential industrial applications. Catalyst preparation NPs of 8.0±0.7-nm CoO x (ref. 22 ) and 6.1±1.0-nm MnO x (ref. 19 ; Supplementary Fig. 5 ), and mesoporous supports [20] , [21] of Co 3 O 4 and MnO 2 ( Supplementary Fig. 6 ) were synthesized according to the literature reports. NP syntheses were carried out using the standard Schlenk techniques. Synthesis of 8-nm Co NPs Oleic acid (150 μl; Aldrich, 99%) was degassed and argon-purged three times in a 250-ml three-neck round-bottom flask fitted with a condenser column. Next 12 ml dichlorobenzene (DCB, Aldrich, anhydrous 99%) was airlessly transferred into the flask and the temperature was raised to 169 °C (5 °C min −1 ). Finally, 0.444 g Co 2 (CO) 8 (Strem Chemicals, stabilized with 1–5% hexanes) dissolved in 3 ml DCB was injected into the flask using a 50-ml airtight syringe. The reaction was allowed to proceed for 20 min. After the heater was turned off, 13 ml DCB was poured into the flask, and the colloidal suspension was allowed to cool down. The Co NPs were collected by centrifugation and re-dispersed in 10 ml chloroform for further use. Synthesis of 6-nm MnO NPs For the synthesis of Mn-oleate, 7.92 g MnCl 2 ·4H 2 O (40 mmol, Aldrich 98%) and 24.36 g sodium oleate (80 mmol, Tokyo Chemical Industry, 95%) were injected into a mixture of 30 ml of ethanol, 40 ml of deionized H 2 O and 70 ml n-hexane at 70 °C under magnetic stirring. The mixture was allowed to react for 4 h. The solution of Mn-oleate (that is, organic phase) was collected by using a separation funnel, and the aqueous phase (that is, NaCl solution) was discarded. The Mn-oleate salt was collected by using a rotatary evaporator. To synthesize 6-nm MnO NPs, 1.24 g Mn-oleate ( ∼ 2 mmol) was dissolved in 10 g of 1-octadecene (Aldrich, 98%) in a 50-ml round-bottom flask. After degasing at 70 °C for 1 h, temperature of the flask was ramped to 280 °C (1.9 °C min −1 ). The colour of the solution changed from pink to transparent and finally to pale green when temperature reached 280 °C. The reaction was allowed to reflux for 10 min. The MnO NPs were collected by centrifugation and re-dispersed in chloroform for further use. m-Co 3 O 4 and MnO 2 For a typical synthesis of KIT-6, 27 g of P123 (Sigma-Aldrich, Mw= ∼ 5,800) and 43.5 ml of concentrated HCl were dissolved in 980 ml of water. Then, 33.3 ml of n -butanol was added to the solution at 35 °C with vigorous stirring. After 1 h of stirring, 58 g of tetraethyl orthosilicate (Sigma-Aldrich, 99%) was added to the solution while vigorously stirring at 35 °C for 24 h. The mixture was reacted hydrothermally at 40 °C overnight. The filtered solid was dried and calcined at 550 °C for 6 h. To prepare m-Co 3 O 4 or -MnO 2 , 4.7 g of cobalt (II) nitrate hexahydrate (Co(NO 3 ) 2 ·6H 2 O, Sigma-Aldrich, 98%) or 4.0 g of manganese (II) nitrate tetrahydrate (Mn(NO 3 ) 2 ·4H 2 O, Sigma-Aldrich, 97%) dissolved in 8 ml of water was mixed with 4 g of KIT-6 and 50 ml of toluene at 65 °C. After evaporating the toluene and water, the solid was collected and calcined at 300 °C for 6 h in air. Then, an aqueous solution of 2 M NaOH at 60 °C was added to the solid and the solution was shaken to dissolve the silica template. After centrifugation, the precipitate was washed with deionized water. The washing with 2 M NaOH solution and deionized water was repeated three times to remove the silica template completely. m-Co 3 O 4 or MnO 2 replicas were obtained after three cycles of centrifugation and drying. MnO x /m-Co 3 O 4 catalysts A hybrid oxide catalyst comprising MnO x NPs supported on m-Co 3 O 4 was prepared by the capillary inclusion method. Briefly, a desired amount of colloidal MnO x NPs dispersed in chloroform were diluted with 40 ml of n -hexane and mixed with m-Co 3 O 4 . The mixture was sonicated for 3 h at room temperature. The precipitate was collected by centrifugation and washed with a 50:50 v/v mixture of acetone and ethanol five times. The precipitated solid was dried at 80 °C overnight. Previously, we reported that 10 nm CoO x NPs gave rise to the highest CO 2 hydrogenation activity measured over SiO 2 and TiO 2 supports [22] . Nonetheless, 8 nm CoO x NPs have been chosen for this study as a compromise between optimal activity and comparable particle sizes with MnO x NPs that could be synthetically produced. MnO x NPs were supported in m-Co 3 O 4 or m-SiO 2 (MCF-17) denoted as MnO x /m-Co 3 O 4 and MnO x /m-SiO 2 , respectively. Similarly, CoO x NPs were supported in m-MnO 2 or m-SiO 2 (MCF-17) and labelled as CoO x /m-MnO 2 and CoO x /m-SiO 2 , respectively. Surface-area measurements Brunauer-Emmett-Teller (BET) measurements were performed using a Micromeritics ASAP 2020 porosity instrument. BET surface areas were evaluated for the reduced catalysts as well as the pristine catalysts ( Supplementary Table 1 ). The reductive treatment was carried out in 1 bar H 2 for 1 h and at three temperatures: 250, 350 and 450 °C, separately. Evaluation of catalyst loading Zeiss Ultra55 analytical scanning electron microscopy equipped with an EDAX energy-dispersive spectrometer (EDS) was employed to determine the loadings of CoO x /m-MnO 2 and MnO x /m-Co 3 O 4 catalysts. An average of 10 EDS spectra that were taken at both low magnification ( × 300) and high magnification ( × 25,000) were used to calculate the % wt. Co (CoO x /m-MnO 2 and CoO x /m-SiO 2 ) or Mn (MnO x /m-Co 3 O 4 and MnO x /m-SiO 2 ), shown in Supplementary Table 1 . Turnovers were calculated from BET surface areas and known surface packing densities of cubic (space group Fm-3m) CoO and MnO. STEM/EELS studies and analysis Jeol 2100F TEM was used in the scanning mode along with a GIF Tridiem Gatan EELS and an Inca EDS. STEM/EELS studies were performed at an accelerating voltage of 120 kV. Convergence and collection semi-angles were 12 mrad. Full-width half-maximum of the zero loss peak was measured to be ∼ 1 eV at a dispersion of 0.2 eV per channel (2,048 channels). Elemental analysis was carried out by using the standard Gatan/EELS software assuming a power law for the pre-edge background and the hydrogenic model for quantification. The results of quantification are tabulated in Supplementary Table 1 . For the analysis of Mn and Co L edge spectra, a slightly modified procedure developed by Pennycook and co-workers [23] was employed, as illustrated in Supplementary Fig. 7 . Following the pre-edge removal, two step functions, one at each of the L 3 and L 2 edges and of the same amplitude as the edge jump were further subtracted from the data. Least-squares fittings of the L 3 and L 2 white line peaks were carried out by constraining amplitude, loss energy and full-width half-maximum. Refined amplitudes were used to calculate the L 3 /L 2 ratios. STEM/EDS studies were carried out at an accelerating voltage of 200 kV with the holder tilted 15° to the EDS detector. XAS studies and analysis Synchrotron-based XAS was performed on beamlines 6.3.1.2 (ISAAC) and 8.0.1 (wet-RIXS) at the Advanced Light Source at the Lawrence Berkeley National Laboratory. Co and Mn L XAS spectra were collected in the ∼ 10 −8 -mbar base pressure in the TEY mode by measuring the compensating electron flow from earth to sample. The X-ray absorption spectra were first normalized relative to X-ray flux. Next, the pre-edge background was removed, and the reduced data were normalized relative to step edge. Linear combination fittings of the reference spectra to the sample were carried out to obtain relative atomic fractions ( Supplementary Figs 1, 8 and 9 ). Catalytic tests and conditions Catalytic testing was performed using a home-built plug-flow reactor operating in a temperature range of 200–450 °C and a pressure range of 1–6 bar. The catalysts were conditioned at 350 °C first in flowing 50 vol.% dry air in balance He followed by flowing 20 vol.% H 2 in balance He for 1 h each, separated by a 15 min He flush (50 sccm) between the two steps. Select catalysts were separately reduced at 250, 450 as well as 350 °C ( Supplementary Fig. 3b ). The catalytic hydrogenation of CO 2 was carried out at 6 bar of CO 2 :H 2 :He (6.4:20.7:16.7) flowing at 42 sccm (delivered via carefully calibrated MKS mass flow controllers). The reactants and products, separated via SS columns packed with 5-A˚ molecular sieves, were monitored online using a HP 5890 II gas chromatograph equipped with a thermal conductivity detector and a flame ionization detector. Catalyst charges of 2–100 mg were used for catalyst testing. All catalysts were evaluated in the low-conversion regime of 3–7%, and select catalysts were also run in the high-conversion regime (that is, limited by reverse water gas shift reaction) of 50–60% range. Space velocity was kept constant at ∼ 150,000 h −1 by mixing catalysts with m-SiO 2 (MCF-17) in the reactor bed. The catalytic reaction was carried out for more than 15 h and the reported turnovers and yields were calculated after this stability run. NPs of CoO x and MnO x supported in m-SiO 2 and pure mesoporous oxides were used as control catalysts ( Supplementary Figs 3 and 4 ). Chemical and morphological properties of the as-made catalysts The as-synthesized catalysts were characterized using STEM and XAS. STEM/EDS phase spectra indicated that Mn was well dispersed over a Co matrix, while STEM/EELS point spectra, taken at 11 edge positions on various oxide grains, showed average O/(Co+Mn) and Mn/(Co+Mn) ratios of 1.4 and 0.04, respectively (see Fig. 2 ). Furthermore, XAS TEY revealed Mn (that is, Mn L) with (II), (III) and (IV) redox centres and Co (that is, Co L) in a pure spinel-ordered Co 3 O 4 phase for the MnO x /m-Co 3 O 4 catalyst ( Supplementary Fig. 8 ). The initial chemical composition of the MnO x NPs was determined as MnO:Mn 3 O 4 :MnO 2 (0.3:0.5:0.2) with a very small concentration of Mn 2 O 3 ( ∼ 0.01). For the CoO x /m-MnO 2 catalyst, the STEM/EDS results, likewise, pointed to a uniformly dispersed Co over ordered mesoporous Mn matrix in the Supplementary Figs 6b and 10 , while STEM/EELS point spectra, taken at 10 edge positions on various oxide grains, showed average O/(Co+Mn) and Co/(Co+Mn) ratios of 1.6 and 0.03, respectively (see Supplementary Fig. 11 ). Moreover, XAS TEY showed the MnO 2 phase with a small fraction of Mn 3 O 4 ( ∼ 0.1) and a mixture of metallic Co, cubic CoO and spinel-ordered Co 3 O 4 with fractions of 0.05:0.65:0.3, respectively, in the Supplementary Fig. 9 . How to cite this article: Li, C.-S. et al . High-performance hybrid oxide catalyst of manganese and cobalt for low-pressure methanol synthesis. Nat. Commun . 6:6538 doi: 10.1038/ncomms7538 (2015).